Mutualistic mycorrhiza-like symbiosis in the most ancient group of land plants Over 35 years ago, it was hypothesized that mutualistic symbiotic soil fungi assisted land plants in their initial colonization of terrestrial environments. This important idea has become increasingly established with palaeobotanical and molecular investigations dating the interactions between arbuscular mycorrhizal fungi (AMF) and land plants to at least 400 Ma, but the functioning of analogous partnerships in 'lower' land plants remains unknown. In this study, we show with multifactorial experiments that colonization of a complex thalloid liverwort, a member of the most ancient extant clade of land plants, with AMF significantly promotes photosynthetic carbon uptake, growth and asexual reproduction. Plant fitness increased through fungal-enhanced acquisition of phosphorus and nitrogen from soil, with each plant supporting 100–400 m of AMF mycelia. A simulated CO 2 -rich atmosphere, similar to that of the Palaeozoic when land plants originated, significantly amplified the net benefits of AMF and likely selection pressures for establishment of the symbiosis. Our analyses provide essential missing functional evidence supporting AMF symbionts as drivers of plant terrestrialization in early Palaeozoic land ecosystems. The colonization of the land by terrestrial plants approximately 450 million years ago (Ma) was one of the most far-reaching chapters in Earth's history [1] . In proposing that symbiotic soil fungi assisted plants in 'greening the Earth', Pirozynski and Malloch [2] boldly conjectured that such 'mycorrhizal associations' were mutualistic, with the fungus gaining photosynthate in return for supplying the host plant with mineral nutrients and water. Although this widely accepted paradigm is consistent with fossil [3] , [4] and molecular clock [5] , [6] evidence, our understanding of arbuscular mycorrhizal fungi (AMF) in 'lower' land plants is confined to structural analyses of the cellular-scale interface between fungal endosymbionts and 'lower' land plants [7] , [8] , [9] and DNA identification of their fungal partners [8] , [9] , [10] , [11] , [12] , [13] . Critically, we lack experimental evidence for the functional nature of the intimate association between early land plant clades and the Glomeromycota, the ancient phylum of fungi that exclusively forms the ancestral arbuscular mycorrhizal (AM) symbiosis [14] . Moreover, arbuscules, the defining structures of symbiotic carbon-for-nutrient exchange in AM, although widely found in AMF associations with complex thalloid liverworts [8] , [9] are atypical or absent in some evolutionarily ancient 'lower' land plant associations with Glomeromycotean fungi [7] . This raises intriguing questions as to their functional equivalence to the AM symbiosis in autotrophic higher plants [12] , [14] , [15] , [16] . In this study, we report experiments directly addressing the hypothesis [2] that a mutually beneficial symbiosis with AM fungi assisted the terrestrialization of multicellular green plants (embryophytes) over 400 Ma. Our multifactorial experiments focus on a widely distributed complex thalloid liverwort Marchantia paleacea in the class Marchantiopsida [17] that diverged approximately 370 Ma [18] . Liverworts are supported as the most basal land plant group by evidence from both molecular phylogenies [19] , [20] and fossils [21] , [22] . Experiments were conducted with the dominant haploid gametophyte phase of the life cycle. We generated even-aged M. paleacea for the experiments by propagating field populations originating from soil in cool temperate cloud forests, Veracruz, Mexico. AMF colonization was manipulated by collecting non-infected vegetative propagules (gemmae) and growing them either in AMF-free soil on their own, or adjacent to AMF-colonized gametophytes to ensure the formation of their normal symbiotic associations. This approach allowed us to resolve the long-standing technical challenge of establishing populations of liverworts with and without their native AMF associations, as the fungal symbionts are difficult to isolate and cannot be maintained in pure culture. Because liverworts possess rhizoids, rather than 'true' roots, we designate their AM associations as 'mycorrhiza-like' [15] (AML). In our experimental design, gametophytes with mycorrhiza-like association (AML) and without (non-mycorrhizal, NM) were grown at ambient CO 2 (400 p.p.m.) or elevated CO 2 (1,500 p.p.m., 3.75×ambient) concentrations, the latter representative of the Palaeozoic [23] . At each atmospheric CO 2 concentration, plants were grown with available nitrogen and phosphorus either at a low concentrations (4.8±0.12 and 2.3±0.12 μg g −1 , respectively) or medium concentrations (23.0±0.9 and 4.8±1.0 μg g −1 , respectively). These soil nutrient supply rates were chosen to represent the oligotrophic conditions of the early Palaeozoic terrestrial environment [24] , and more nutrient-rich microhabitats [25] . Our results establish that AMF form mutualistic symbiosis in a thalloid liverwort, a member of the most ancient group of land plants, in which this symbiosis is assumed to be a basal trait [9] , [19] . The symbiosis improved plant growth and fitness through enhancing nutrient uptake, especially phosphorus, and the plant supported enhanced AM fungal biomass in soil. The benefits to the host plant are strongly amplified by elevated atmospheric CO 2 concentrations, which would have promoted the symbiosis in the initial phase of plants 'greening the Earth' in the early Palaeozoic. Evidence of host plant infection by fungal endosymbionts Sectioning of thalli of field populations, and AML individuals used in the experiments, revealed the cortical parenchyma to be heavily colonized by aseptate fungal hyphae, with a distinctive red pigmentation to the cell walls ( Fig. 1a )—a feature absent in NM-'control' thalli ( Fig. 1b ). Fungal hyphae colonized the thallus tissue directly and through smooth rhizoids. The fungal partner forms extensive coils in some of the cells, many of which formed arbuscules ( Fig. 1c ), in agreement with earlier observations on M. paleacea [9] and other species of Marchantia [8] , [9] . The endosymbionts of M. paleacea were revealed using DNA sequencing to be members of Glomus group Ab ( Fig. 1d ). Previous studies of Marchantia foliacea sampled from eight sites in New Zealand found all plants colonized by Glomus group A fungi, and about half the samples colonized by Glomus group Ab fungi [8] . 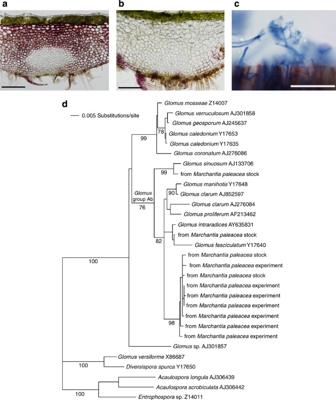Figure 1: LiverwortM. paleaceagametophyte colonized by glomeromycete endosymbionts. (a) Thallus cross-section showing cells with red pigmented walls colonized by glomeromycete fungi, below the green photosynthetic tissue and above the rhizoids extending below the central axis, (b) uncolonized thallus lacking red pigmentation and (c) arbuscule released from the edge of a longitudinal section through the fungal-colonized part of the thallus, stained with Trypan blue. (d) Neighbour-joining distance tree of fungi based on 960 bp of 5′ 18S nuclear ribosomal DNA sequences. Bootstrap percentages are shown below branches.Glomusgroup Ab was rooted with members ofGlomusgroup C (Glomus versiforme,Diversispora spurca) and Acaulosporaceae (Acaulosporaspp.,Entrophosporasp.). Scale bar in (a) and (b) is 250 μm and in (c) is 50 μm. Figure 1: Liverwort M. paleacea gametophyte colonized by glomeromycete endosymbionts. ( a ) Thallus cross-section showing cells with red pigmented walls colonized by glomeromycete fungi, below the green photosynthetic tissue and above the rhizoids extending below the central axis, ( b ) uncolonized thallus lacking red pigmentation and ( c ) arbuscule released from the edge of a longitudinal section through the fungal-colonized part of the thallus, stained with Trypan blue. ( d ) Neighbour-joining distance tree of fungi based on 960 bp of 5′ 18S nuclear ribosomal DNA sequences. Bootstrap percentages are shown below branches. Glomus group Ab was rooted with members of Glomus group C ( Glomus versiforme , Diversispora spurca ) and Acaulosporaceae ( Acaulospora spp., Entrophospora sp.). Scale bar in ( a ) and ( b ) is 250 μm and in ( c ) is 50 μm. Full size image Increased host plant photosynthesis Liverworts forming symbiotic partnerships with AMF exhibited significantly enhanced photosynthetic carbon gain, as revealed by gas exchange measurements of net CO 2 assimilation rates at growth ( A op ) and saturating ( A sat ) irradiances ( Fig. 2 ). We analysed their dependence on the treatments using a linear mixed effects model [26] that included a random effect for plant, and the effects of AMF, CO 2 concentration and irradiance (likelihood ratio test, P <0.0001 for all terms) ( Fig. 2 ). AML individuals exhibited significantly enhanced A op and A sat compared to NM plants, under both ambient and elevated CO 2 ( P <0.001) ( Fig. 2 ), with no significant effect of soil nutrient status (likelihood ratio test, P >0.06). There was no evidence for interactions between AML status, soil nutrients, CO 2 or irradiance (likelihood ratio test, P >0.1 for all terms), indicating that the treatments affected A op and A sat in the same manner. Carbon dioxide fertilization of A sat allows AML liverworts to be more successful across a broader range of light environments. The lack of downregulation of A sat at high CO 2 ( Fig. 2 ) suggests that the below-ground AMF network provided a carbon sink for the additional photosynthate, alleviating potential end-product inhibition [27] . In this respect, comparatively slow-growing mycorrhizal liverworts appear to behave similarly to AM-vascular land plants [28] under high CO 2 . 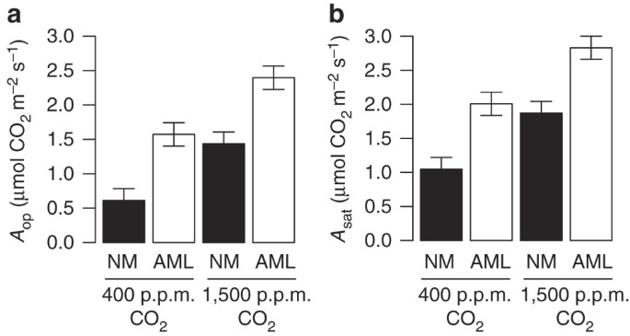Figure 2: Arbuscular mycorrhizal fungi enhance liverwort photosynthetic carbon gain. Steady-state operational net CO2assimilation rates (Aop) of arbuscular mycorrhiza-like (AML) or non-mycorrnizal (NM)M. paleaceagrown at (a) ambient CO2(400 p.p.m.) and elevated CO2(1,500 p.p.m.), measured at the respective treatment CO2. (b) light-saturated CO2assimilation rates (Asat) of AML and NM plants from the same treatments as in (a). All values are means±s.e. Rates ofAopandAsatwere measured on a randomly selected subset of three plants in each treatment and were highly correlated (r2=0.78,n=24,P<0.00001). Analysis with a linear mixed effects model26, which included a random effect for plant, identified significant effects of mycorrhiza, growth CO2concentration and irradiance (likelihood ratio test,P<0.0001 for all terms). Figure 2: Arbuscular mycorrhizal fungi enhance liverwort photosynthetic carbon gain. Steady-state operational net CO 2 assimilation rates ( A op ) of arbuscular mycorrhiza-like (AML) or non-mycorrnizal (NM) M. paleacea grown at ( a ) ambient CO 2 (400 p.p.m.) and elevated CO 2 (1,500 p.p.m. ), measured at the respective treatment CO 2 . ( b ) light-saturated CO 2 assimilation rates ( A sat ) of AML and NM plants from the same treatments as in ( a ). All values are means±s.e. Rates of A op and A sat were measured on a randomly selected subset of three plants in each treatment and were highly correlated ( r 2 =0.78, n =24, P <0.00001). Analysis with a linear mixed effects model [26] , which included a random effect for plant, identified significant effects of mycorrhiza, growth CO 2 concentration and irradiance (likelihood ratio test, P <0.0001 for all terms). Full size image Increased host plant growth Positive effects of AML status on photosynthetic CO 2 fixation of the liverwort translated directly into significantly enhanced gametophyte growth ( Fig. 3 ). We characterized the growth of all 48 individuals using a four-parameter logistic model with nonlinear mixed effects [26] ; this closely fitted the data (see Supplementary information ) and allowed us to estimate the treatment effects after accounting for differences in plant size at the beginning of the experiment. Arbuscular mycorrhiza-like status, soil nutrient supply (likelihood ratio tests, P <0.00001 in both cases) and CO 2 enrichment (likelihood ratio test, P <0.03) all significantly enhanced the final biomass of the plants ( Fig. 3 ). No significant interactions between AML status, soil nutrients and CO 2 were detected ( P >0.1 in all cases). AMF colonization and soil nutrients individually increased the final biomass by a factor of 1.7 (95% confidence interval 1.5–1.9), whereas CO 2 enrichment effects were smaller, increasing final biomass by a factor of 1.2 (95% confidence interval 1.03–1.34). The effects of AMF, greater soil nutrient supply and elevated CO 2 were additive and, in combination, dramatically increased final biomass ( ∼ 3.4-fold). Much of this is driven by AMF and nutrients (2.9-fold relative to uninfected plants with no added nutrients and ambient CO 2 ). In effect, AML plants on soils of low nutrient status, representing oligotrophic early Palaeozoic surface environments [24] , attained a similar biomass to NM plants on more nutrient-rich soil ( Fig. 3 ). 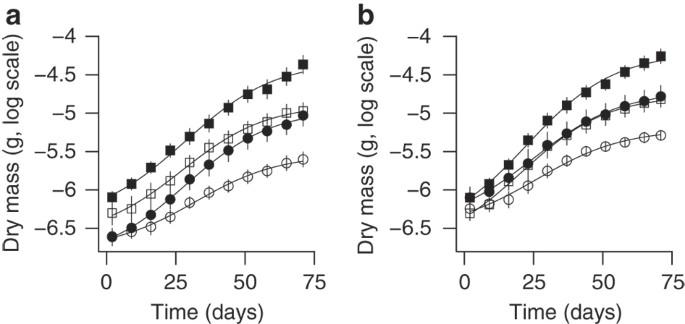Figure 3: Arbuscular mycorrhizal fungi enhance liverwort primary production. Fitted logistic growth curves (mean±s.e.) of (a) arbuscular mycorrhiza-like (AML, ▪) and non-mycorrnizal (NM, □)M. paleaceadry mass with medium soil nutrient supply, and mycorrhiza-like (AML, •) and non-mycorrhizal (NM,○)M. paleaceawith low soil nutrient supply at ambient CO2(400 p.p.m.). (b) As in (a) but for liverworts grown in elevated CO2(1,500 p.p.m.). AML symbiosis, soil nutrient status (likelihood ratio tests,P<0.00001 in both cases) and CO2enrichment (likelihood ratio test,P<0.03) all significantly enhanced the final biomass of the plants. No significant interactions between AML status, soil nutrients and growth CO2were detected (P>0.1 in all cases).n=6 gametophytes per treatment, 48 in total. Figure 3: Arbuscular mycorrhizal fungi enhance liverwort primary production. Fitted logistic growth curves (mean±s.e.) of ( a ) arbuscular mycorrhiza-like (AML, ▪) and non-mycorrnizal (NM, □) M. paleacea dry mass with medium soil nutrient supply, and mycorrhiza-like (AML, •) and non-mycorrhizal (NM, ○ ) M. paleacea with low soil nutrient supply at ambient CO 2 (400 p.p.m.). ( b ) As in ( a ) but for liverworts grown in elevated CO 2 (1,500 p.p.m.). AML symbiosis, soil nutrient status (likelihood ratio tests, P <0.00001 in both cases) and CO 2 enrichment (likelihood ratio test, P <0.03) all significantly enhanced the final biomass of the plants. No significant interactions between AML status, soil nutrients and growth CO 2 were detected ( P >0.1 in all cases). n =6 gametophytes per treatment, 48 in total. Full size image Increased host plant fitness Benefits of AMF to the host liverworts extended to the greater production of asexual reproductive propagules, with AML plants producing 78% of all the gemmae ( Supplementary Table S1 ). The overall frequency of gemmae production by AML plants (across CO 2 and nutrient treatments) was significantly higher than for NM controls ( χ 2 =12.9, 1 d.f., P <0.001). Allometric analyses indicated that gemmae production on the final census (day 71) increased with thallus biomass, and was described by a highly significant (likelihood ratio test, P <0.00001) generalized linear model assuming a Poisson distribution for gemmae production ( Fig. 4 ). Elevated CO 2 increased gemmae production over and above its effect on biomass (likelihood ratio test, P <0.0003) ( Fig. 4 ), so that at a given plant size, those in elevated CO 2 produced 3.83 times more gemmae per gram of thallus dry mass (95% confidence interval 1.66–8.94). Although the confidence intervals on this estimate are wide, even the lower bound suggests that CO 2 enrichment increased gemmae production per unit thallus mass by 66%. AML symbiosis and elevated CO 2 , therefore, strongly would promote the asexual dispersal of the host plant and colonization of new habitats. Parallel benefits to the formation of reproductive structures have been inferred for more recently evolved jungermannialean (leafy) liverworts forming endosymbiotic partnerships with higher fungal groups [29] . 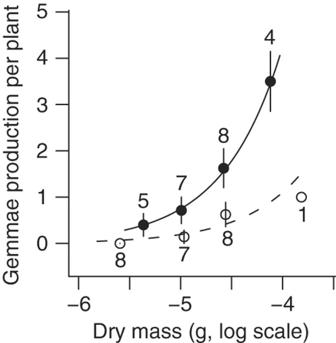Figure 4: Asexual reproduction increases with liverwort size. Relationship between thallus mass (M) and gemmae production (G) for ambient (○, dashed line) and elevated (•, solid line) CO2grown plants. All values are means±s.e. Numbers indicate number of plants. The dashed fitted line is for ambient CO2plants,G=exp(7.1[1.8]+1.7[0.4]×M) and the solid fitted line is for elevated CO2plants,G=exp(8.4[1.7]+1.7[0.4]×M), figures in square parentheses are standard errors. The effects of thallus mass and growth CO2concentration is highly significant (likelihood ratio tests,P<0.00001 andP<0.0003, respectively), but the interaction between thallus mass and CO2was not significant (likelihood ratio test,P>0.8). Figure 4: Asexual reproduction increases with liverwort size. Relationship between thallus mass ( M ) and gemmae production ( G ) for ambient ( ○ , dashed line) and elevated (•, solid line) CO 2 grown plants. All values are means±s.e. Numbers indicate number of plants. The dashed fitted line is for ambient CO 2 plants, G =exp(7.1[1.8]+1.7[0.4]×M) and the solid fitted line is for elevated CO 2 plants, G =exp(8.4[1.7]+1.7[0.4]×M), figures in square parentheses are standard errors. The effects of thallus mass and growth CO 2 concentration is highly significant (likelihood ratio tests, P <0.00001 and P <0.0003, respectively), but the interaction between thallus mass and CO 2 was not significant (likelihood ratio test, P >0.8). Full size image Increased soil nitrogen and phosphorus uptake AM fungal hyphae are highly adapted to mobilize and translocate phosphorus from soils [16] . Consequently, a primary benefit to plants hosting AM fungi is the provision of phosphorus that would otherwise be inaccessible to rhizoids due to depletion zones immediately surrounding these structures that result from uptake and slow diffusive replacement of phosphate ions [16] . Tissue chemistry analyses support a similar role for AM fungi in liverwort nitrogen and phosphorus nutrition. Treatment effects on total phosphorus uptake by M. paleacea paralleled those on final biomass, with total phosphorus uptake significantly (likelihood ratio test, P <0.00001) increased by 70% in AML plants at ambient CO 2 and elevated CO 2 within a given nutrient treatment, indicating that AMF increased the capture and transfer of soil phosphorus to host gametophytes. The constancy of thallus phosphorus concentrations, which were not significantly affected by AML infection status, nutrient supply or growth CO 2 (2.22±0.06 μg phosphorus per mg dry mass, mean±s.e., three-way analysis of variance, P >0.08 for main effects and interactions), indicates that the growth of the liverwort was primarily constrained by its rate of phosphorus uptake. These results for total phosphorus and thallus phosphorus concentrations in a liverwort growing on soil-based substrate, and colonized by natural populations of AMF symbionts from the field, are reinforced by findings from in vitro experiments with the thalloid liverwort Lunularia [30] . Our findings confirm that limited phosphorus availability constrains the growth of the liverwort, and the primary benefit and function of its AML association is to enhance the capture of this element to increase biomass, growth and reproduction. This is consistent with the hypothesis [2] that the evolution of AM was vital for the successful colonization of land by plants through assisting the acquisition of phosphorus from nutrient-poor soils. Colonization by AMF significantly increased thallus nitrogen concentration by 30% over asymbiotic plants (three-way analysis of variance, F 1,18 =55.9, P <0.002); 12.8±0.55 compared with 9.9±0.59 μg per mg dry mass, respectively. This benefit may enhance the production of photosynthetic pigments and enzymes, both of which require significant nitrogen investment. It may also enable the production of more gemmae, and increase their nutrient deposits. The AML association increased the total amount of nitrogen captured more than four-fold under elevated CO 2 , suggesting direct involvement of the AMF in nitrogen uptake from soil, as in higher plants [16] . Critically, our results suggest that the high CO 2 atmosphere of the Palaeozoic [23] lowered the relative 'carbon-for-nutrient cost' to plants of AMF compared with current situation at ambient CO 2 , thereby providing enhanced benefits from improved phosphorus and nitrogen nutrition, as evidenced by enhanced biomass, nutrient uptake and photosynthetic efficiency ( Figs 2 and 3 ). Evidence for mutualism To determine whether the AMF-liverwort symbiosis is mutualistic, with demonstrable benefits to the fungal partners, we measured hyphal lengths under AML M. paleacea , corrected for background values from NM plants. This indicated that individual adult thalli supported 100–400 m of AMF mycelium (274.9±53.1, mean±s.e. ), and provides clear evidence for receipt of photosynthate by the fungus because AMF lack the saprotrophic abilities to use soil organic carbon sources [16] . These hyphae gave an additional absorptive surface area for nutrient uptake of 20–185 cm 2 for each plant (80.5±10.6, mean±s.e.). Neither the length of hyphae nor their area per plant was significantly influenced by nutrients or CO 2 (two-way analysis of variance, P >0.4 for all main effects and the interaction), but given the large inter-plant variability larger sample sizes may be required to resolve such effects. We have demonstrated the existence of a mutualistic symbiosis between glomeromycete endosymbiotic fungi and an extant non-vascular plant lineage occupying the most basal node on the land plant phylogenetic tree [19] , [20] . Recent molecular evidence indicates vertical inheritance of the same suite of genes for mycorrhiza formation from gametophytes of liverworts to sporophytes of vascular plants [31] . This provides compelling support for AMF associations in liverworts being a basal and ancestral trait, despite the plants now associating with more recently evolved fungal clades, such as the Glomus Ab group [32] . The genetic machinery underlying mycorrhizal symbiosis is highly conserved across widely divergent plant taxa, and the evidence of its vertical inheritance supports the view that land plants evolved from a single common mycorrhizal ancestor [31] . Furthermore, the Marchantiales, together with the other basal liverwort groups Haplomitriales and Treubiales, appear to be restricted to forming symbiotic associations with the basal phylum of symbiotic fungi of land plants (Glomeromycota) [15] , which occur in 80–100% of over 30 extant species examined in these families to date [9] . These twin lines of evidence indicate that extant basal land plant glomeromycotean fungal partnerships provide analogues for the Palaeozoic situation [1] , [2] , [5] , [15] , [31] . One intriguing aspect of the AML fungal associations in M. paleacea is its association with fungi in the Glomus group Ab. This is the same fungal group found with high specificity both in the sister species M. foliacea [8] , and forming intergenerational mycelial networks [12] between the haploid gametophyte and diploid sporophyte stages of the 'lower' tracheophyte clubmosses ( Lycopodium and Huperzia [10] ), and the 'lower' ferns Botrychium [11] and Psilotum [13] . Of the fungal sequences currently available in GenBank, the Glomus colonizing M. paleacea in our experiments were most similar to those sequenced from Psilotum nudum [13] , a tracheophyte with sporophytes that by convergent evolution show close morphological similarities to early vascular land plant fossils [3] , [4] but are of more recent origin; the Psilotaceae is the sister group to the Ophioglossales in the monilophytes, which includes horsetails and ferns [33] . The genera Lycopodium [10] , [34] , Botrychium [10] , [35] , Ophioglossum [36] and Psilotum [13] , [37] all include species with gametophytes that are achlorophyllous. These plants are mycoheterotrophic parasites of Glomus group Ab fungal partners, which obtain their carbon by forming mycorrhizal associations with adjacent sporophytes or other autotrophic plants [12] . Many mycoheterotrophic higher plants, including Voyria and Voyriella in the Dicotyledonae and Arachnitis in the Monocotyledonae, show high specificity to clades of the Glomus Ab group that they parasitise [38] . Fine-level co-evolutionary analysis within Afrothismia , a genus of mycoheterotrophic higher plant, and its AMF partners [39] provided insight into the mechanistic basis of its extreme fidelity to a clade of Glomus group A fungi, and its descendant lineages, that has persisted over the past 50 Ma. In this association, speciation in Afrothismia tracked the much older evolutionary history of the Glomeromycotean fungi that diverged from a basal clade in Glomus group A approximately 220 Ma [39] providing further support for the vertical transmission of specific mycorrhization genes [31] . The potential specificity to Glomus Ab fungi seen in Marchantia liverworts, and in the gametophytes and sporophytes of 'lower' tracheophytes, may therefore have arisen by the evolutionary tracking of AMF fungal phylogeny as seen in Afrothismia . By always associating with a narrow clade of fungi with high specificity, these far more ancient plant groups could have tracked the evolutionary pathway from a basal common ancestral Glomus to the Glomus Ab group. This suggestion would seem at least as plausible as multiple horizontal host switching [15] , [32] by the diverse group of 'lower' and higher plants that are specialized on Glomus Ab group, a mechanism for which is unknown. Host shifting from tracheophytes to liverworts is established in some of the more recently derived families of simple thalloid and leafy liverworts [40] . Some of these have lost their ancestral glomeromycete associations and replaced them with ascomycete and basidiomycete fungal associations that probably invaded these liverworts from symbiotic associations already established with higher plants [40] . In providing the first evidence of mutualistic symbiotic associations between a thalloid liverwort and glomeromycotean fungal partners, we establish functional equivalence to the AM mycorrhiza of higher plants [3] , [4] , [14] , [15] . The formation of arbuscules in Marchantian thalloid liverworts [8] , [9] is consistent with their Glomus Ab group AMF associations providing mutualistic carbon-for-nutrient exchange. It contrasts with the parasitism of AMF fungi in the same group by mycoheterotrophic gametophytes of 'lower' tracheophytes, and mycoheterotrophic higher plants, in both of which arbuscules are typically absent [34] , [35] , [36] , [37] . Further studies are now required to establish the functioning of AML associations in simple thalloid liverworts in the genera Treubia and Haplomitrium , as these have atypical arbuscule-like structures, with sparse branching and terminal swellings [7] , similar to those found in the photosynthetic sporophytes of the simple fern Ophioglossum [41] . Our experiments establish essential missing functional evidence supporting the 35-year-old conjecture [2] that an ancient widespread and mutualistic symbiotic partnership between AMF and basal land plants assisted the colonization of the continents. Furthermore, we extend this bold hypothesis by demonstrating that the high CO 2 atmosphere of the Palaeozoic [23] amplified the benefits of AMF by increasing the growth-limiting rates of phosphorus uptake in a rootless 'lower' land plant and its reproductive output. It therefore likely created a uniquely strong selection pressure favouring the establishment of mycorrhiza-like partnerships with AMF in the gametophyte-dominant phase of early land plants [3] , [4] , whose subsequent evolution fundamentally changed the ecology and climate of the planet [1] . Growth and tissue chemistry analyses AML and NM plants were grown in controlled environment chambers (Conviron) with day–night temperatures of 18 and 15 °C, respectively, a 12-h day length, 80–85% relative humidity (RH) and 20 μmol m −2 s −1 photosynthetically active radiation (PAR). Plants were watered and misted on a daily basis with reverse osmosis water. Following establishment, from gemmae (see main text), NM and AML gametophytes were transferred to individual large (10 cm diameter×15 cm) pots containing a mixture of washed sand and either 8 or 32% commercial compost (John Innes Seed Compost), giving 4.8±0.12 and 2.3±0.12 μg g −1 available nitrogen and phosphorus, respectively (low nutrient) and 23.0±0.9 and 4.8±1.0 μg g −1 available nitrogen and phosphorus (medium nutrient), as determined by standard methods [42] . Mean (±s.e.) pH=7.3±0.04, no significant difference between treatments. The growth of each individual ( n =6 per treatment, 48 total) was tracked non-destructively every week with digital photography (Nikon, D80) and the images analysed for surface area with image analysis software (Image J, NIH, http://rsbweb.nih.gov/ij ). The presence/absence of AMF in AML and NM plants, respectively, at the end of the experiment was confirmed by hand sectioning and direct microscopic observation of the thallus tissue for fungal hyphae. Tissue phosphorus and nitrogen was determined with standard methods [42] , and hyphal lengths with extraction and staining techniques followed by grid-line intercept counting on a gridded membrane [43] . Hyphal lengths were determined from soil cores (10 mm diameter, 60 mm depth) removed from beneath the plants. Total AMF lengths, and absorptive surface areas per plant, were calculated as the difference between those of AML and NM plants for a given treatment, with measured bulk densities of the low nutrient (8% compost) and medium nutrient (32% compost) substrates of 1.49 and 1.43 g cm −3 and a rooting volume of 576 cm 3 . Detailed observations of the hyphae confirmed the typical anatomical features of AMF, including angular projections and the general absence of septa, or where these were present the septa were simple [16] . Hyphal surface area was calculated as that of a cylinder with a typical AMF width of 6 μm [16] . Molecular identification of fungal endosymbionts We extracted genomic DNA from stock and experimental thallus fragments approximately 2 mm long using established methods [44] , with a purification step using GeneClean (QBioGene). We then amplified (PicoMaxx, Stratagene or JumpStart, Sigma), cloned (TOPO TA, Invitrogen) and sequenced (BigDye v.3 on ABI3730 Genetic Analyzer, Applied Biosystems) portions of fungal ribosomal RNA genes using nested specific primer sets [45] and the fungal primers ITS1F [44] and ITS4 [46] . Because only glomeromycete Glomus group Ab DNA sequences were retrieved, we then amplified and sequenced a 960-bp fragment of small subunit rDNA with primers NS1 [46] and AM1 [47] . Phylogenetic analyses were conducted with PAUP version 4.0b10 (Phylogenetic Analysis Using Parsimony, Sinauer Associates). Representative DNA sequences are deposited in GenBank under accession numbers FR690120, FR690121 and FR690122. Gas exchange measurements Net CO 2 assimilation rates ( A ) were measured on thallus tissue after 70 days with an infra-red gas exchange analyzer (LiCor-6400, LI-COR Biosciences) by placing the tissue within a standard leaf cuvette modified with nylon strands to suspend the tissue above the thermocouple. All measurements were carried out at the growth CO 2 concentration (400 or 1,500 p.p.m.) at 18 °C (i.e., day-time growth temperature), 80–85% RH, and with a tissue surface area of at least 1–2 cm 2 . Steady-state measurements were carried out at the growth irradiance (20 μmol m −2 s −1 PAR) and the light-saturating irradiance, as determined from A -PAR curves to be 100 μmol PAR m −2 s −1 . During A measurements, thallus tissue remained hydrated and turgid, enclosed within the cuvette at 80–85% RH; liverworts can generally tolerate 30% moisture loss before A rates are affected [48] . Growth analyses We used area and dry mass after drying at 70 °C for 48 h data from the final harvest to construct a regression model for converting thallus area to mass. There were no effects of treatment ( P >0.4 in all cases), so the final regression model was where M is mass in grams and A is area in cm 2 , figures in parentheses are standard errors, this model was highly significant ( P <0.00001) and accounted for 83% of the variance in log mass ( Supplementary Fig. S1 ). Note the relationship is isometric (slope not significantly different from unity) suggesting that the thallus thickness does not vary with thallus area or treatment. Area measurements were carried out on 11 dates and these converted to mass using Equation (1). Plots of the time series of masses ( Supplementary Fig. S2 ) show there is considerable between plant differences related to initial mass, and these differences are consistent throughout the experiments. To account for the consistent between-individual differences, we used a nonlinear mixed effects model [26] . We characterized the growth curve of each individual using a four-parameter logistic model of the form where m P , i ( t ) is log mass of the i th individual at time t , m max, i is the asymptotic mass, m min, i is the minimum mass, t 0, i is the time when plant mass is midway between m max, i and m min, i , and k i a growth rate parameter (large values corresponding to rapid growth). The growth curves were fitted as nonlinear mixed effects models using the nlme package [26] in R ( http://www.r-project.org/ ) [49] and we followed their recommendations for model simplification. The final fitted model has correlated, individual-specific random effects for m min, i , m max, i and t 0, i , and the asymptotic mass, m max, i , included fixed effects for AMF infection status, nutrients and CO 2 . Note that by allowing the initial size to vary between individuals we can estimate the treatment effects allowing for the differences in plant size at the beginning of the experiment. The fixed effects of AML association and nutrient status were highly significant (likelihood ratio test, P <0.00001), whereas the effect of CO 2 enhancement was marginally significant (likelihood ratio test, P <0.03). We also explored the model with interactions between the treatments, but the interactions never entered the model significantly (likelihood ratio test, P >0.1 in all cases). Fitted individual-specific curves are shown in Supplementary Figure S3 . We calculated the average growth curves for each treatment combination by averaging the individual-specific growth curves. Accession numbers: Representative DNA sequences are deposited in GenBank under accession numbers FR690120–FR690122. How to cite this article: Humphreys, C.P. et al . Mutualistic mycorrhiza-like symbiosis in the most ancient group of land plants. Nat. Commun. 1:103 doi: 10.1038/ncomms1105 (2010).